Total synthesis and antiviral activity of indolosesquiterpenoids from the xiamycin and oridamycin families Indolosesquiterpenoids are a growing class of natural products that exhibit a wide range of biological activities. Here, we report the total syntheses of xiamycin A and oridamycins A and B, indolosesquiterpenoids isolated from Streptomyces . Two parallel strategies were exploited to forge the carbazole core: 6π-electrocyclization/aromatization and indole C2–H bond activation/Heck annulation. The construction of their trans -decalin motifs relied on two diastereochemically complementary radical cyclization reactions mediated by Ti(III) and Mn(III), respectively. The C23 hydroxyl of oridamycin B was introduced by an sp 3 C–H bond oxidation at a late stage. On the basis of the chemistry developed, the dimeric congener dixiamycin C has been synthesized for the first time. Evaluation of the antiviral activity of these compounds revealed that xiamycin A is a potent agent against herpes simplex virus–1 (HSV-1) in vitro . Indolosesquiterpenoids have attracted increasing attention from chemical and biosynthetic perspectives [1] , [2] , [3] , [4] , [5] , [7] ; however, their biological activities are yet to be systematically explored through chemical synthesis [8] , [9] , [10] , [11] , [12] , [13] , [14] . Xiamycin A ( 1 , Fig. 1 ), isolated independently from Streptomyces species by Hertweck [15] , [16] , [17] , [18] and Zhang [19] , [20] , [21] , displays selective anti-HIV activity. The naturally occurring antibiotics oridamycins A and B ( 2 and 3 ) share a similar scaffold to that of 1 , though with the opposite stereochemistry at quaternary C16 (ref. 22 ). Several congeners of 1 were also identified from the same species, including the C6–N1′ dimer dixiamycin C ( 4 ), the C11–C12 bond oxidized and ring-expanded oxiamycin ( 5 ) and a putative biosynthetic precursor, indosespene ( 6 ) [17] , [18] , [19] , [20] , [21] . Considerable efforts have been made towards revealing the biogenesis of this class of natural products, including the elucidation of the relevant gene clusters and enzymes [17] , [18] , [19] , [20] . The chemical synthesis of these compounds [13] , [14] may help further the understanding of the biosynthetic relationships within this indolosesquiterpenoid family, as well as the discovery of their unknown biological activities. Very recently, Baran et al . [13] disclosed the first total synthesis of xiamycin A ( 1 ) and dixiamycin B. 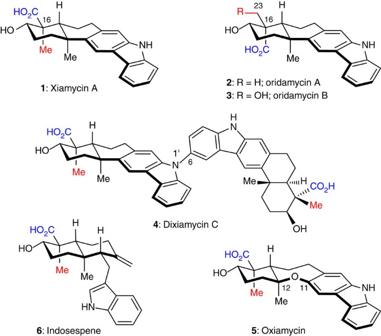Figure 1: The structures of representative natural products from the xiamycin and oridamycin families. The two families share a similar scaffold but differ in the C16 stereochemistry. Indosespene (6) is a putative biosynthetic precursor of xiamycin A (1). Figure 1: The structures of representative natural products from the xiamycin and oridamycin families. The two families share a similar scaffold but differ in the C16 stereochemistry. Indosespene ( 6 ) is a putative biosynthetic precursor of xiamycin A ( 1 ). Full size image In this paper, we report the total syntheses of xiamycin A, oridamycins A and B, dixiamycin C ( 1 – 4 ) and indosespene ( 6 ). The syntheses of 2 – 4 were accomplished for the first time. A 6π-electrocyclization strategy and an oxidative Heck annulation strategy were developed for assembling the carbazole scaffold. The antiviral properties of the synthetic natural products were evaluated in vitro , and 1 exhibits potent inhibitory activity against herpes simplex virus–1 (HSV-1). Retrosynthetic analysis The synthetic challenge of the xiamycin and oridamycin families may be separated into two distinct problems, namely the stereocontrolled assembly of the trans -decalin motif bearing the C16 quaternary centre and the construction of the carbazole core. Inspired by the structural correlation between xiamycin A ( 1 ) and indosespene ( 6 ), our retrosynthetic analysis of 1 ( Fig. 2 ) began with a disconnection at the C2–C21 bond. A 6π-electrocyclization [23] (path a) and a Heck-type annulation [24] , [25] , [26] , [27] , [28] , [29] (path b) were envisioned as two alternatives to forge the carbazole motif. The former draws on our recent syntheses of tubingensin A and daphenylline [30] , [31] , while the latter relies on activation of the indole C2–H bond by palladium. Correspondingly, triene ( 7 ) and indosespene ester ( 8 ) are considered as the key intermediates for the two strategies. These functionalized decalin systems are expected to arise from a cascade cyclization of dienylepoxide precursors, such as 9 and 10 . This type of radical cyclization may be initiated by reduction of the epoxide by a Ti(III) species [32] , [33] , [34] , [35] , [36] , [37] , [38] , [39] , [40] , [41] , [42] , [43] , [44] , [45] , [46] , [47] , although, to our knowledge, α,β-epoxy esters/ketones have not been fully explored as the substrates for such cyclization [14] , [48] . Notably, Cuerva and coworkers [49] disclosed that enol radicals derived from α,β-unsaturated ketones inhibit the cyclization reaction. The stereochemical outcome of the cyclization cascade (including the stereochemistry at C16) would be determined by the chirality and geometry of the precursor, which may allow a convenient access to oridamycins A and B ( 2 and 3 ) from an alternative precursor. Successful execution of the route outlined above would also be anticipated to provide access to indosespene ( 6 ) and dixiamycin C ( 4 ) through minor modifications. 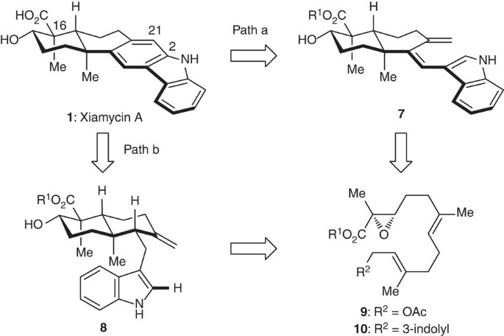Figure 2: Two retrosynthetic analyses of xiamycin A. One (path a) features a 6π-electrocyclization/aromatization strategy, and the other (path b) involves an indole C2–H bond activation/Heck annulation strategy. The devised strategies are anticipated to be applicable to the synthesis of other members from the xiamycin and oridamycin families. Figure 2: Two retrosynthetic analyses of xiamycin A. One (path a) features a 6π-electrocyclization/aromatization strategy, and the other (path b) involves an indole C2–H bond activation/Heck annulation strategy. The devised strategies are anticipated to be applicable to the synthesis of other members from the xiamycin and oridamycin families. Full size image The 6π-electrocyclization/aromatization approach Fig. 3 illustrates the 6π-electrocyclization/aromatization approach for the synthesis of xiamycin A ( 1 ). Starting from optically active epoxide 11 (96% ee) [50] , a sequence of 2-azaadamantane N -oxyl (AZADO) oxidation [51] , [52] and esterification led to compound 12 in 76% overall yield. On the basis of seminal work on the Ti(III)-catalysed bioinspired epoxypolyene cyclization by Cuerva and Oltra [38] , [39] , [40] , [41] , we investigated the cyclization of the α,β-epoxy ester 12 . Under the optimized conditions [Cp 2 TiCl 2 (20 mol%), Mn, i Pr 2 NEt, TMSCl], the desired trans -decalin 13 was obtained as a single diastereomer. TBS protection followed by acetyl deprotection gave 14 (44% yield for the three steps), which was subjected to a sequence of DMP oxidation, Grignard addition (with reagent 15 ) [30] , and dehydration (MsCl/ i Pr 2 NEt) to furnish triene 16 in 75% overall yield. On microwave irradiation (120 °C, air), 16 underwent a thermal 6π-electrocyclization and a subsequent aromatization to generate carbazole 17 (80% yield). Similarly, when using Grignard reagent 18 with a bromine substituent, we readily obtained compound 19 via the corresponding triene 20 . This bromocarbazole served as an appropriate substrate for the crucial C–N bond formation in our dixiamycin C synthesis ( vide infra ). Desulfonylation of 17 followed by TMSE deprotection of the resulting compound 21 afforded xiamycin A ( 1 ) in a good overall yield, the structure of which was confirmed by X-ray crystallographic analysis ( Fig. 4 ). 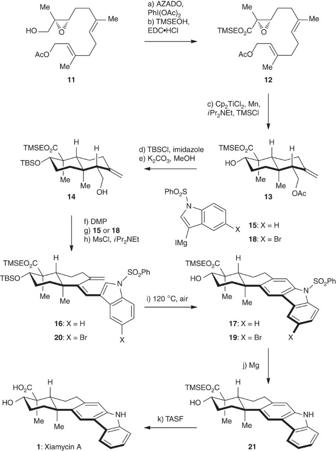Figure 3: The 6π-electrocyclization/aromatization approach towards the total synthesis of xiamycin A. Reagents and conditions: (a) AZADO (5 mol%), PhI(OAc)2(3.0 eq), CH2Cl2, 22 °C, 6 h; (b) TMSEOH (1.2 eq), EDC·HCl (1.1 eq), 4-DMAP (1.0 eq), CH2Cl2, 22 °C, 5 h, 76% (two steps); (c) Cp2TiCl2(20 mol%), Mn (8.0 eq),iPr2NEt (6.0 eq), TMSCl (5.0 eq), THF, 22 °C, 4 h; (d) TBSCl (1.2 eq), imidazole (1.5 eq), DMF, 22 °C, 10 h; (e) K2CO3(1.0 eq), MeOH, 22 °C, 3 h, 44% (3 steps); (f) DMP (1.5 eq), CH2Cl2, 22 °C, 30 min; (g)15or18(3.0 eq), THF, 22 °C, 40 min; (h) MsCl (1.2 eq),iPr2NEt (1.5 eq), CH2Cl2, 0 °C, 1 h, 75% for16(three steps), 71% for20(three steps); (i) air, DMSO, 120 °C, 2 h, 80% for17, 76% for19; (j) Mg (2.0 eq), MeOH, 22 °C, 1 h, 98%; (k) TASF (2.0 eq), DMF, 50 °C, 95%. Figure 3: The 6π-electrocyclization/aromatization approach towards the total synthesis of xiamycin A. Reagents and conditions: (a) AZADO (5 mol%), PhI(OAc) 2 (3.0 eq), CH 2 Cl 2 , 22 °C, 6 h; (b) TMSEOH (1.2 eq), EDC·HCl (1.1 eq), 4-DMAP (1.0 eq), CH 2 Cl 2 , 22 °C, 5 h, 76% (two steps); (c) Cp 2 TiCl 2 (20 mol%), Mn (8.0 eq), i Pr 2 NEt (6.0 eq), TMSCl (5.0 eq), THF, 22 °C, 4 h; (d) TBSCl (1.2 eq), imidazole (1.5 eq), DMF, 22 °C, 10 h; (e) K 2 CO 3 (1.0 eq), MeOH, 22 °C, 3 h, 44% (3 steps); (f) DMP (1.5 eq), CH 2 Cl 2 , 22 °C, 30 min; (g) 15 or 18 (3.0 eq), THF, 22 °C, 40 min; (h) MsCl (1.2 eq), i Pr 2 NEt (1.5 eq), CH 2 Cl 2 , 0 °C, 1 h, 75% for 16 (three steps), 71% for 20 (three steps); ( i ) air, DMSO, 120 °C, 2 h, 80% for 17 , 76% for 19 ; ( j ) Mg (2.0 eq), MeOH, 22 °C, 1 h, 98%; (k) TASF (2.0 eq), DMF, 50 °C, 95%. 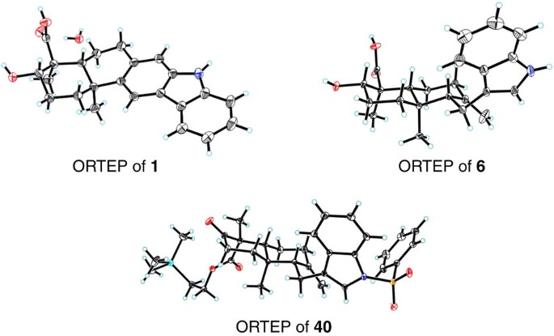Figure 4: ORTEP drawings of compounds1,6and40. Non-hydrogen atoms are shown as 30% ellipsoids. The stereochemical outcomes of the radical cyclization cascades are unambiguously confirmed. Full size image Figure 4: ORTEP drawings of compounds 1 , 6 and 40 . Non-hydrogen atoms are shown as 30% ellipsoids. The stereochemical outcomes of the radical cyclization cascades are unambiguously confirmed. Full size image The mechanism of the cascade cyclization is postulated in Fig. 5 . The epoxide C16–O bond is reductively cleaved by the Ti(III) species to generate 22 , which triggers two sequential cyclization reactions, and the resulting radical 23 could undergo a mixed disproportionation [53] to give the intermediate 24 with an exocyclic C=C bond. In fact, two side reactions occurred: 1, over reduction of 22 to the corresponding enolate [48] followed by β-elimination to form an α,β-unsaturated ester; 2, hydrogen transfer to 23 to form the saturated derivative of 24 . Organic bases had subtle influence on these undesired reactions [54] , and i Pr 2 NEt was found to suppress the latter effectively in our case. Considering the challenges for the acid-promoted epoxy polyene cyclization, such as the preference to the formation of products with tri-/tetrasubstituted olefins and difficulty generating carbocations with electron-withdrawing substituents, this radical chemistry offers a useful and complementary route for preparing functionalized sesquiterpenoid synthons. 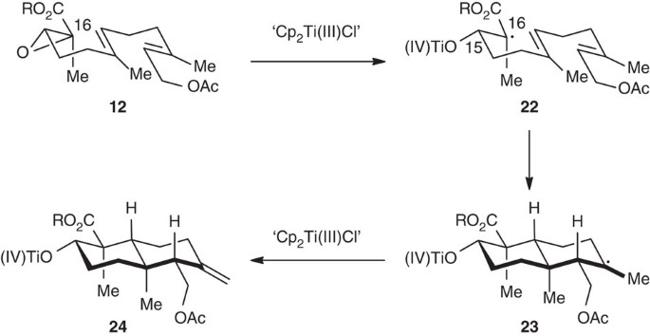Figure 5: A postulated mechanism of the Ti(III)-mediated radical cyclization. The epoxy ester serves as a suitable substrate for this reaction. Thetrans-decalin system with an equatorial alkoxycarbonyl and an exocyclic methylene groups is obtained. Figure 5: A postulated mechanism of the Ti(III)-mediated radical cyclization. The epoxy ester serves as a suitable substrate for this reaction. The trans -decalin system with an equatorial alkoxycarbonyl and an exocyclic methylene groups is obtained. Full size image We then focused on the synthesis of oridamycin A bearing an axial carboxylic substituent on C16 ( Fig. 6 ). The cis -epoxy analogue of 12 was first prepared and subjected to the Ti(III) conditions. However, the compound 13 with an equatorial carboxylic substituent was detected as the major product, presumably due to the fast rotation of the C15–C16 bond to adopt the sterically favoured conformation ( Fig. 5 ) for the cyclization. Thus, we made recourse to a mechanistically different oxidative radical cyclization mediated by Mn(III) [55] , [56] , [57] , [58] , [59] using β-ketoester 25 (ref. 56 ) as a substrate. Treatment with Mn(OAc) 3 /Cu(OAc) 2 in DMSO effected the radical cyclization with an acceptable yield of decalin 26 (48%, a single diastereomer detected). This compound was subjected to a sequence similar to that described above to afford triene 27 with good overall efficiency, via the intermediacy of aldehyde 28 . Under thermal conditions (120 °C) and in presence of air, 27 was converted to carbazole 29 (83% yield) in one pot. Sequential ketone reduction (NaBH 4 ) and desulfonylation (Mg/MeOH) provided compound 30 in 83% overall yield. Final TMSE deprotection led to the completion of the first synthesis of (±)-oridamycin A ( 2 ). 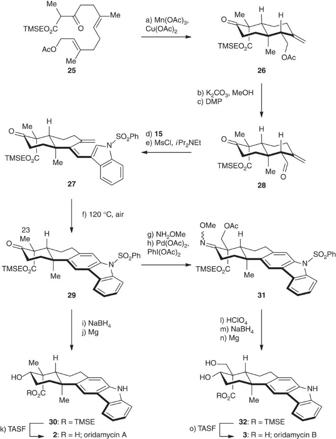Figure 6: The 6π-electrocyclization/aromatization approach towards the total syntheses of oridamycins A and B. Reagents and conditions: (a) Mn(OAc)3·2H2O (2.0 eq), Cu(OAc)2·H2O (1.0 eq), DMSO, 22 °C, 12 h, 48%; (b) K2CO3(1.5 eq), MeOH, 22 °C, 3 h; (c) DMP (2.0 eq), CH2Cl2, 22 °C, 30 min, 92% (two steps); (d)15(3.0 eq), THF, 22 °C, 40 min; (e) MsCl (1.2 eq),iPr2NEt (1.5 eq), CH2Cl2, 0 °C, 1 h, 74% (2 steps); (f) air, DMSO, 120 °C, 2 h, 83%; (g) NH2OMe·HCl (2.0 eq), pyridine, 22 °C, 2 h, 94%; (h) Pd(OAc)2(20 mol%), PhI(OAc)2(1.0 eq), Ac2O/AcOH (1:1), 110 °C, 1 h, 82%; (i) NaBH4(3.0 eq), MeOH, 0 °C, 30 min; (j) Mg (8.0 eq), MeOH, 22 °C, 1 h, 83% (two steps); (k) TASF (2.0 eq), DMF, 50 °C, 92%; (l) aq. HClO4(6.0 M)/acetone (1:3), 22 °C, 12 h; (m) NaBH4(3.0 eq), MeOH, 0 °C, 30 min, 62% (2 steps); (n) Mg (8.0 eq), MeOH, 22 °C, 1 h, 90%; (o) TASF (2.0 eq), DMF, 50 °C, 91%. Figure 6: The 6π-electrocyclization/aromatization approach towards the total syntheses of oridamycins A and B. Reagents and conditions: (a) Mn(OAc) 3 ·2H 2 O (2.0 eq), Cu(OAc) 2 ·H 2 O (1.0 eq), DMSO, 22 °C, 12 h, 48%; (b) K 2 CO 3 (1.5 eq), MeOH, 22 °C, 3 h; (c) DMP (2.0 eq), CH 2 Cl 2 , 22 °C, 30 min, 92% (two steps); (d) 15 (3.0 eq), THF, 22 °C, 40 min; (e) MsCl (1.2 eq), i Pr 2 NEt (1.5 eq), CH 2 Cl 2 , 0 °C, 1 h, 74% (2 steps); (f) air, DMSO, 120 °C, 2 h, 83%; (g) NH 2 OMe·HCl (2.0 eq), pyridine, 22 °C, 2 h, 94%; (h) Pd(OAc) 2 (20 mol%), PhI(OAc) 2 (1.0 eq), Ac 2 O/AcOH (1:1), 110 °C, 1 h, 82%; (i) NaBH 4 (3.0 eq), MeOH, 0 °C, 30 min; (j) Mg (8.0 eq), MeOH, 22 °C, 1 h, 83% (two steps); (k) TASF (2.0 eq), DMF, 50 °C, 92%; (l) aq. HClO 4 (6.0 M)/acetone (1:3), 22 °C, 12 h; (m) NaBH 4 (3.0 eq), MeOH, 0 °C, 30 min, 62% (2 steps); (n) Mg (8.0 eq), MeOH, 22 °C, 1 h, 90%; (o) TASF (2.0 eq), DMF, 50 °C, 91%. Full size image We accomplished the synthesis of oridamycin B for the first time by adjusting the C23 oxidation state of 29 ( Fig. 6 ), taking advantage of the neighbouring ketone carbonyl group. O -Methyloxime formation afforded the substrate suitable for a directed C–H bond oxidation, and Sanford’s conditions [Pd(OAc) 2 (20 mol%), PhI(OAc) 2 ] [60] , [61] were effective to give the desired acetate 31 with good overall efficiency. It should be noted that stoichiometric Pd-mediated Csp 3 –H bond oxidation reactions have been exploited in terpenoid synthesis [41] , [62] , [63] . Deprotection of the oxime and acetate, followed by reduction and desulfonylation, afforded diol 32 with acceptable overall efficiency. Removal of TMSE with TASF provided (±)-oridamycin B ( 3 ) in 91% yield. The spectroscopic data of the synthetic samples of oridamycins A and B matched those reported for the natural products. The C–H bond activation/Heck annulation approach The second approach to xiamycin A ( 1 ) fulfilled the strategy of indole C2–H activation/Heck-type annulation ( Fig. 7 ). Stille coupling [64] of 12 with N -Boc-3-(tributylstannyl)indole 33 [65] followed by deprotection of Boc [66] provided a fully functionalized precursor 34 (66% overall yield), which underwent a Ti(III)-catalysed radical cyclization under the same conditions as above to give decalin 35 as a single diastereomer in 60% yield [39] . In the presence of Pd(OAc) 2 and p -benzoquinone at 50 °C (refs 28 , 29 ), 35 was converted to carbazole 21 in 81% yield, presumably through the devised oxidative Heck/aromatization sequence. TMSE deprotection of 35 and 21 with TASF then afforded indosespene ( 6 ) and xiamycin A ( 1 ), respectively. The structure of 6 was verified by X-ray crystallographic analysis ( Fig. 4 ). 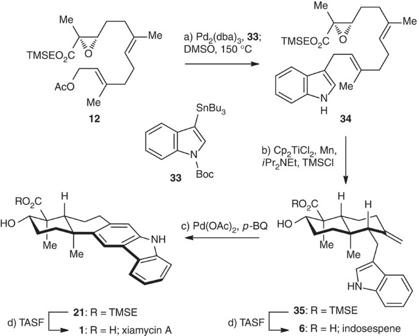Figure 7: The oxidative Heck annulation approach towards the total synthesis of xiamycin A. Reagents and conditions: (a) Pd2(dba)3(5 mol%), LiCl (3.0 eq),33(2.0 eq), DMF, 80 °C, 2 h, then DMSO, 150 °C, 30 min, 66%; (b) Cp2TiCl2(20 mol%), Mn (8.0 eq),iPr2NEt (6.0 eq), TMSCl (5.0 eq), THF, 22 °C, 4 h, 60%; (c) Pd(OAc)2(20 mol%),p-benzoquinone (2.0 eq), AcOH/toluene (1:4), 50 °C, 2 h, 81%; (d) TASF (2.0 eq), DMF, 50 °C, 95% for1, 91% for6. Figure 7: The oxidative Heck annulation approach towards the total synthesis of xiamycin A. Reagents and conditions: (a) Pd 2 (dba) 3 (5 mol%), LiCl (3.0 eq), 33 (2.0 eq), DMF, 80 °C, 2 h, then DMSO, 150 °C, 30 min, 66%; (b) Cp 2 TiCl 2 (20 mol%), Mn (8.0 eq), i Pr 2 NEt (6.0 eq), TMSCl (5.0 eq), THF, 22 °C, 4 h, 60%; (c) Pd(OAc) 2 (20 mol%), p -benzoquinone (2.0 eq), AcOH/toluene (1:4), 50 °C, 2 h, 81%; (d) TASF (2.0 eq), DMF, 50 °C, 95% for 1 , 91% for 6 . Full size image The above strategy was further applied to alternative syntheses of oridamycins A and B ( Fig. 8 ). In this case, an indole-containing β-ketoester 36 was employed as the substrate for the Mn(III) mediated cyclization. N -Sulfonylation of 3-geranylindole 37 ( ref. [67] ; NaOH, PhSO 2 Cl) and subsequent allylic oxidation (SeO 2 , t BuOOH) gave alcohol 38 in 78% overall yield, which underwent bromination (Et 3 N, MsCl; LiBr) followed by alkylation with the dianion generated from β-ketoester 39 (KH, then BuLi) to furnish 36 (80% yield for the two steps). Under the similar conditions used for the cyclization of compound 25 ( Fig. 6 ), decalin 40 was obtained in 52% yield as a single detectable diastereomer. Its C16 stereochemistry was secured by X-ray crystallographic analysis ( Fig. 4 ). Desulfonylation (Mg/MeOH, 96% yield) and subsequent oxidative Heck annulation ( vide supra ) afforded carbazole 41 (65% yield), which was subjected to a two-step sequence of ketone reduction and TMSE deprotection to give (±)-oridamycin A ( 2 ). Sanford Csp 3 –H bond oxidation was exploited again for the synthesis of oridamycin B from 41 ; deactivation of the carbazole motif with an electron-withdrawing N -protecting group was required. Thus, 41 was subjected to NH 2 OMe condensation and Boc protection to afford the oxidation precursor. The same conditions [Pd(OAc) 2 (20 mol%), PhI(OAc) 2 ] as used before delivered acetate 42 smoothly (67% yield for the three steps). Global deprotection of the oxime, acetyl and Boc groups under acidic conditions followed by reduction of the exposed carbonyl group furnished the late intermediate 32 in 54% overall yield, which was converted to (±)-oridamycin B ( 3 ) through the removal of TMSE group. 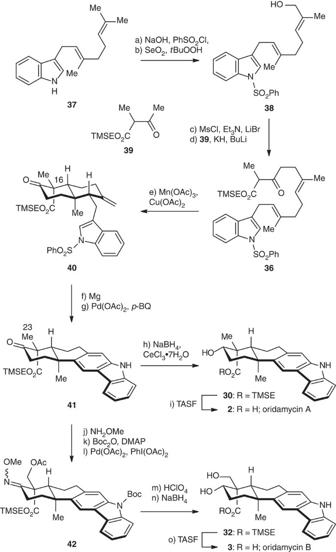Figure 8: The oxidative Heck annulation approach towards the total syntheses of oridamycins A and B. Reagents and conditions: (a) PhSO2Cl (2.0 eq), Bu4NBr (10 mol%), aq. NaOH (50 wt%)/toluene (1:2), 22 °C, 3 h; (b) SeO2(20 mol%),tBuOOH (2.0 eq), CH2Cl2, 0 °C, 10 h, 78% (two steps); (c) Et3N (1.5 eq), MsCl (1.2 eq), LiBr (5.0 eq), THF, 0 °C, 30 min; (d)39, (1.0 eq), KH (1.2 eq), BuLi (1.2 eq), THF/HMPA (5:1), 0 °C, 3 h, 80% (two steps); (e) Mn(OAc)3·2H2O (2.0 eq), Cu(OAc)2·H2O (1.0 eq), DMSO, 22 °C, 12 h, 52%; (f) Mg (3.0 eq), NH4Cl (1.2 eq), MeOH, 22 °C, 1 h, 96%; (g) Pd(OAc)2(20 mol%),p-benzoquinone (2.5 eq), AcOH/toluene (1:4), 50 °C, 2 h, 65%; (h) NaBH4(3.0 eq), CeCl3·7H2O (3.0 eq), MeOH, 0 °C, 30 min; (i) TASF (2.0 eq), DMF, 50 °C, 2 h, 85% (two steps); (j) NH2OMe·HCl (2.0 eq), pyridine, 22 °C, 2 h, 93%; (k) Boc2O (2.0 eq), 4-DMAP (2.0 eq), THF, 22 °C, 1 h, 89%; (l) Pd(OAc)2(20 mol%), PhI(OAc)2(1.1 eq), Ac2O/AcOH (1:1), 110 °C, 1 h, 81%; (m) aq. HClO4(6.0 M)/acetone (1:3), 22 °C, 8 h; (n) NaBH4(3.0 eq), MeOH, 0 °C, 30 min, 54% (two steps); (o) TASF (2.0 eq), DMF, 50 °C, 2 h, 91%. Figure 8: The oxidative Heck annulation approach towards the total syntheses of oridamycins A and B. Reagents and conditions: (a) PhSO 2 Cl (2.0 eq), Bu 4 NBr (10 mol%), aq. NaOH (50 wt%)/toluene (1:2), 22 °C, 3 h; (b) SeO 2 (20 mol%), t BuOOH (2.0 eq), CH 2 Cl 2 , 0 °C, 10 h, 78% (two steps); (c) Et 3 N (1.5 eq), MsCl (1.2 eq), LiBr (5.0 eq), THF, 0 °C, 30 min; (d) 39 , (1.0 eq), KH (1.2 eq), BuLi (1.2 eq), THF/HMPA (5:1), 0 °C, 3 h, 80% (two steps); (e) Mn(OAc) 3 ·2H 2 O (2.0 eq), Cu(OAc) 2 ·H 2 O (1.0 eq), DMSO, 22 °C, 12 h, 52%; (f) Mg (3.0 eq), NH 4 Cl (1.2 eq), MeOH, 22 °C, 1 h, 96%; (g) Pd(OAc) 2 (20 mol%), p -benzoquinone (2.5 eq), AcOH/toluene (1:4), 50 °C, 2 h, 65%; (h) NaBH 4 (3.0 eq), CeCl 3 ·7H 2 O (3.0 eq), MeOH, 0 °C, 30 min; (i) TASF (2.0 eq), DMF, 50 °C, 2 h, 85% (two steps); (j) NH 2 OMe·HCl (2.0 eq), pyridine, 22 °C, 2 h, 93%; (k) Boc 2 O (2.0 eq), 4-DMAP (2.0 eq), THF, 22 °C, 1 h, 89%; (l) Pd(OAc) 2 (20 mol%), PhI(OAc) 2 (1.1 eq), Ac 2 O/AcOH (1:1), 110 °C, 1 h, 81%; (m) aq. HClO 4 (6.0 M)/acetone (1:3), 22 °C, 8 h; (n) NaBH 4 (3.0 eq), MeOH, 0 °C, 30 min, 54% (two steps); (o) TASF (2.0 eq), DMF, 50 °C, 2 h, 91%. Full size image The synthesis of dixiamycin C Having synthesized the monomeric natural products, we directed our attention to the synthesis of dixiamycin C ( Fig. 9 ). Starting from coupling partners 19 and 21 , we investigated a variety of conditions for the transition metal promoted C–N bond formation. Buchwald’s protocol [68] [CuI, (±)- 43 , K 3 PO 4 , 110 °C] proved to be optimal to provide dimer 44 . Deprotection of the benzenesulfonyl and TMSE groups furnished dixiamycin C ( 4 ) in a good overall yield, via the intermediacy of 45 . The spectra and physical properties of the synthetic dixiamycin C were consistent with those reported for the natural products. 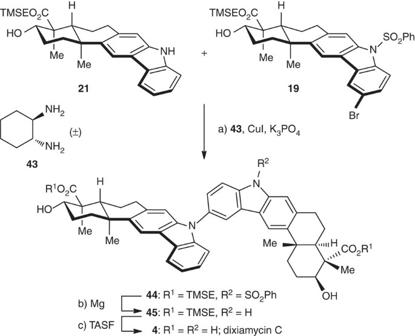Figure 9: Total synthesis of dixiamycin C. Reagents and conditions: (a) CuI (1.5 eq),21(1.0 eq),19(1.5 eq), (±)-43(3.0 eq), K3PO4(7.5 eq), 1,4-dioxane, 110 °C, 12 h; (b) Mg (6.0 eq), MeOH, 22 °C, 1 h, 51% for the two steps; (c) TASF (4.0 eq), DMF, 50 °C, 5 h, 96%. Figure 9: Total synthesis of dixiamycin C. Reagents and conditions: (a) CuI (1.5 eq), 21 (1.0 eq), 19 (1.5 eq), (±)- 43 (3.0 eq), K 3 PO 4 (7.5 eq), 1,4-dioxane, 110 °C, 12 h; (b) Mg (6.0 eq), MeOH, 22 °C, 1 h, 51% for the two steps; (c) TASF (4.0 eq), DMF, 50 °C, 5 h, 96%. Full size image The antiviral activity The activities of synthetic xiamycin A ( 1 ), oridamycins A ( 2 ), dixiamycin C ( 4 ), indosespene ( 6 ) and sespenine [14] , [16] against HSV-1 and hepatitis C virus (HCV) were evaluated. Notably, xiamycin A was reported to possess moderate anti-HIV activity but no significant cytotoxicity against a number of human tumour cell lines [16] , and a structurally relevant carbazole natural product, named tubingensin A, was found to exhibit anti-HSV-1 activity (without details disclosed) [69] . We treated HSV-1 (KOS strain)-infected vero cells with 5.0 and 0.50 μM solutions of the compounds for 20 h and then quantified the infectious HSV-1 titres in the supernatants by using TCID 50 assay [70] . As shown in Fig. 10 , 1 , 4 , 6 and sespenine can suppress HSV-1 propagation in a dose-dependent manner. Notably, xiamycin A ( 1 ) is the most potent compound that reduces >95% of virus propagation at a concentration of 0.50 μM. Indosespene ( 6 ) significantly inhibits HSV-1 propagation at the concentration of 5.0 μM and displays essentially no antiviral activity at the concentration of 0.50 μM. Dixiamycin C ( 4 ) and sespenine show moderate inhibitory activity against HSV-1 at 5.0 μM but no activity at 0.50 μM. For the anti-HCV test (using a replicon assay), only dixiamycin C ( 6 ) exhibited inhibitory activity at a high concentration (50 μM, see Supplementary Fig. 81 ). It should be mentioned that these compounds did not exhibit cytotoxicity against the cells used for both anti-HSV-1 and HCV tests (see Supplementary Fig. 82 ). 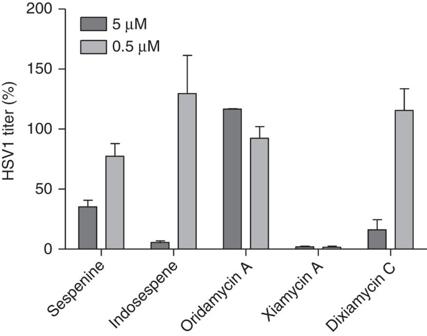Figure 10: Effects of the synthetic compounds on HSV-1 propagation. Vero cells were infected with HSV1 (strain KOS-ATCC VR1493) for 3 h and then treated with different concentrations of compounds for 20 h. HSV-1 in the culture supernatants were then quantified by using TCID50assay. Virus titres were presented as the percentages of the mock DMSO treatment. Data represent means±s.e.m. of six individual infections. Figure 10: Effects of the synthetic compounds on HSV-1 propagation. Vero cells were infected with HSV1 (strain KOS-ATCC VR1493) for 3 h and then treated with different concentrations of compounds for 20 h. HSV-1 in the culture supernatants were then quantified by using TCID 50 assay. Virus titres were presented as the percentages of the mock DMSO treatment. Data represent means±s.e.m. of six individual infections. Full size image We have accomplished the total synthesis of indolosesquiterpenoids xiamycin A, oridamycins A and B, dixiamycin C and indosespene. Two unified strategies for the framework construction and a series of transition-metal-mediated reactions formed the basis of the synthesis. Antiviral tests of the synthetic natural products revealed that xiamycin A exhibits a potent inhibitory activity against HSV-1. General All reactions were carried out under an argon atmosphere with dry solvents under anhydrous conditions, unless otherwise noted. Tetrahydrofuran (THF), toluene and 1,4-dioxane were distilled immediately before use from sodium-benzophenone ketyl. Methylene chloride (CH 2 Cl 2 ), N , N -dimethylformamide (DMF), dimethyl sulfoxide (DMSO), hexamethylphosphoramide (HMPA), triethylamine (Et 3 N), N , N -diisopropylethylamine ( i Pr 2 NEt) and pyridine were distilled from calcium hydride and stored under an argon atmosphere. Methanol (MeOH) was distilled from magnesium and stored under an argon atmosphere. Acetone was dried over drierite and distilled before use. Reagents were purchased at the highest commercial quality and used without further purification, unless otherwise stated. Solvents for chromatography were used as supplied by Titan Chemical. Reactions were monitored by thin layer chromatography (TLC) carried out on S-2 0.25 mm E. Merck silica gel plates (60F-254) using UV light as a visualizing agent and aqueous ammonium cerium nitrate/ammonium molybdate or basic aqueous potassium permanganate as a developing agent. E. Merck silica gel (60, particle size 0.040–0.063 mm) was used for flash column chromatography. Preparative thin layer chromatography separations were carried out on 0.25 or 0.50 mm E. Merck silica gel plates (60F-254). NMR spectra were recorded on Bruker AV-400, DRX-600 or Agilent 500/54/ASP instrument and calibrated by using residual undeuterated chloroform ( δ H =7.26 p.p.m.) and CDCl 3 ( δ C =77.16 p.p.m. ), or undeuterated methanol ( δ H =3.31 p.p.m.) and methanol-d 4 ( δ C =49.00 p.p.m. ), as internal references. IR spectra were recorded on a Thermo Scientific Nicolet 380 FT-IR spectrometer. Melting points (m.p.) are uncorrected and were recorded on a SGW X-4 apparatus. High-resolution mass spectra (HRMS) were recorded on a Bruker APEXIII 7.0 Tesla ESI-FT mass spectrometer. For 1 H and 13 C NMR spectra of compounds, see Supplementary Figs 1–70 . For the comparisons of 1 H and 13 C NMR spectra of the natural and synthetic natural products, see Supplementary Figs 71–80 . For the comparisons of 1 H and 13 C NMR spectroscopic data of the natural and synthetic natural products, see Supplementary Tables 1–10 . For the experimental procedures, and spectroscopic and physical data of compounds, the antiviral assay and cytotoxicity assays, and the crystallographic data of compounds 1 , 6 and 40 , see Supplementary Methods . How to cite this article: Meng, Z. et al . Total synthesis and antiviral activity of indolosesquiterpenoids from the xiamycin and oridamycin families. Nat. Commun. 6:6096 doi: 10.1038/ncomms7096 (2015). Accession codes: The X-ray crystallographic coordinates for structures ( 1 , 6 and 40 ) reported in this Article have been deposited at the Cambridge Crystallographic Data Centre (CCDC), under deposition number CCDC 948203, 949054 and 948503. These data can be obtained free of charge from The Cambridge Crystallographic Data Centre via www.ccdc.cam.ac.uk/data_request/cif.